An instant multi-responsive porous polymer actuator driven by solvent molecule sorption Fast actuation speed, large-shape deformation and robust responsiveness are critical to synthetic soft actuators. A simultaneous optimization of all these aspects without trade-offs remains unresolved. Here we describe porous polymer actuators that bend in response to acetone vapour (24 kPa, 20 °C) at a speed of an order of magnitude faster than the state-of-the-art, coupled with a large-scale locomotion. They are meanwhile multi-responsive towards a variety of organic vapours in both the dry and wet states, thus distinctive from the traditional gel actuation systems that become inactive when dried. The actuator is easy-to-make and survives even after hydrothermal processing (200 °C, 24 h) and pressing-pressure (100 MPa) treatments. In addition, the beneficial responsiveness is transferable, being able to turn ‘inert’ objects into actuators through surface coating. This advanced actuator arises from the unique combination of porous morphology, gradient structure and the interaction between solvent molecules and actuator materials. Adaptive soft matter, such as responsive gels, elastomers, shape memory and electro-active polymers, is attracting burgeoning interest in material science, engineering, medicine and biology [1] , [2] , [3] , [4] , [5] , [6] , [7] , [8] , [9] , [10] , [11] , [12] , [13] , [14] , [15] , [16] , [17] . Fast and robust responsiveness coupled with large-scale displacement are eagerly sought after [18] , which have been the defining feature of biological actuators but missing from synthetic counterparts [19] , [20] , [21] , [22] , [23] , [24] . For example, sea cucumbers can alter the stiffness of their dermis within seconds to obtain survival advantages [19] ; the Venus flytrap can close their leaves in a second for efficient prey capture [20] . On the other hand, the hygroscopic movements of pine cones [24] and ice plant seed capsules [22] , although slower, can function even when the host organisms are dead. Recently, enormous efforts have been paid to these bio-prototypes, with progress being made on responsive nanocomposites and surfaces [3] , energy generators and transducers [25] , [26] , programmable origami [27] , soft robotics [28] , [29] , [30] , smart gels [31] , [32] , [33] and artificial muscles [34] , [35] , [36] . Yet, most of the polymer actuators suffer from the relatively slow and small scale movements; furthermore, they are susceptible to severe circumstances and involve complex preparation such as multi-step lithographic processes [21] , [37] . In this scenario, actuators bearing rapid responsiveness and strong tolerance towards aggressive milieus are highly desirable for promptly and reliably converting external stimuli to mechanical movement. In addition, multi-responsive actuators viable in both the wet and dry states remain a challenge, for example, hydrogel actuators become inactive when dried. To address these requirements, we engineer a novel structural model fostering the ultra-fast and robust actuation movement through the solvent molecule sorption mechanism. Two structural features are essential to this model. First, the major component of the actuator membrane is a cationic poly(ionic liquid) polymer that possesses bulk organic counter anions and can interact with a variety of organic solvent vapours, as will be demonstrated below. Second, the actuator membrane represents a unique synergy of an electrostatic complexation gradient and a porous architecture through the membrane. In this design, the electrostatic complexation provides ionic cross-linking network and structural robustness; the porous structures give rise to a fast responsiveness by accelerating the internal mass transport and the large-scale actuation arising from high compressibility. As such, the mechanical actuation can be instantly triggered by variation of solvent vapour and humidity; the structure also survives very harsh processing steps to prove their wide operation window in various environments. Preparation and characterizations of the porous membrane The porous actuator membrane was prepared from a mixture of solution of a cationic poly(ionic liquid), poly(3-cyanomethyl-1-vinylimidazolium bis(trifuoromethanesulfonyl)imide) (abbreviated as ‘PILTf 2 N’, Tf 2 N denotes the counter anion) and a carboxylic acid-substituted pillar[5]arene (C-pillar[5]arene) that bears 10 acid groups (COOH) ( Supplementary Fig. 1 ). PILTf 2 N and C-pillar[5]arene were first dissolved in dimethyl sulphoxide (DMSO) in a 1:1 molar ratio of the imidazolium cation ring (on PILTf 2 N) to COOH groups (on C-pillar[5]arene). Subsequently the solution was cast on a glass plate and dried at 80 °C for 1 h (please note: the membrane surfaces facing the air and the glass plate are defined as ‘top’ and ‘bottom’ surfaces, respectively). Then the membrane was soaked in aqueous ammonia ( Fig. 1a , left scheme); after 2 h, a free-standing membrane with a scalable size was peeled off from the glass plate and denoted as PILTf 2 N/C-pillar[5]arene ( Supplementary Fig. 2 ). During the soaking step, ammonia diffuses into the membrane from top to bottom, deprotonates the COOH into COO − NH 4 + groups and simultaneously triggers the electrostatic complexation between the negatively charged C-pillar[5]arene with the imidazolium cation from PILTf 2 N. As such, a gradient in the degree of electrostatic complexation (DEC, Supplementary Fig. 3 ) forms along the membrane cross-section ( z direction in Fig. 1a ) because the complexation is coupled to the top-down diffusion of ammonia into the membrane. While the complexation between PILTf 2 N and C-pillar[5]arene is quantitatively accompanied by the release of Tf 2 N counter anions into solution, the DEC is inversely proportional to the Tf 2 N residue in the membrane. Because sulphur exists only in Tf 2 N, its content is a quantitative measure of Tf 2 N concentration. In detail, the Tf 2 N content was found to increase along the top-down direction ( Supplementary Fig. 4 ) and vice versa for the DEC ( Fig. 1e ), that is, the top surface has a lower Tf 2 N content and thus a higher DEC than the bottom. 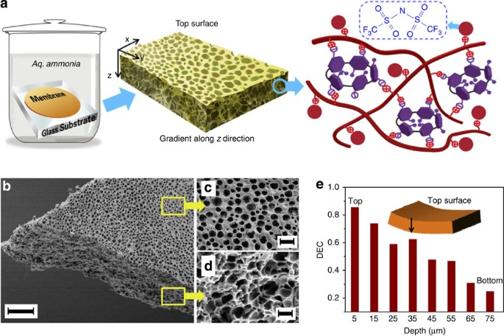Figure 1: Design concept and structure characterizations of the membrane actuator. (a) A scheme illustrating the preparation route (left), porous morphology (middle) and the chemical structure (right) of the PILTf2N/C-pillar[5]arene membrane actuator. On the right: the red line and purple ring represent PILTf2N polymer chains and C-pillar[5]arene molecules, respectively; this cartoon schematises the electrostatic complexation between the imidazolium cations on PILTf2N and the carboxylate anions on C-pillar[5]arene molecules. (b–d) SEMmorphologies of the membrane actuator: general view (b, scale bar (black), 30 μm); top surface (c, scale bar, 3 μm); and cross-section (d, scale bar: 1 μm); (e) the structural gradient of the DEC along the membrane cross-section (top–down direction). The DEC of the membrane is defined as the ratio of the imidazolium units that have electrostatically complexed with COO−groups (on C-pillar[5]arene) to the overall amount of imidazolium units (Supplementary Fig. 3). Experimentally, DEC values at different locations of the membrane are determined by the sulphur content at different locations of the membrane cross-section (Supplementary Fig. 4). Figure 1: Design concept and structure characterizations of the membrane actuator. ( a ) A scheme illustrating the preparation route (left), porous morphology (middle) and the chemical structure (right) of the PILTf 2 N/C-pillar[5]arene membrane actuator. On the right: the red line and purple ring represent PILTf 2 N polymer chains and C-pillar[5]arene molecules, respectively; this cartoon schematises the electrostatic complexation between the imidazolium cations on PILTf 2 N and the carboxylate anions on C-pillar[5]arene molecules. ( b – d ) SEMmorphologies of the membrane actuator: general view ( b , scale bar (black), 30 μm); top surface ( c , scale bar, 3 μm); and cross-section ( d , scale bar: 1 μm); ( e ) the structural gradient of the DEC along the membrane cross-section (top–down direction). The DEC of the membrane is defined as the ratio of the imidazolium units that have electrostatically complexed with COO − groups (on C-pillar[5]arene) to the overall amount of imidazolium units ( Supplementary Fig. 3 ). Experimentally, DEC values at different locations of the membrane are determined by the sulphur content at different locations of the membrane cross-section ( Supplementary Fig. 4 ). Full size image The membrane network is shown to be stable in common organic solvents because electrostatic complexation is characteristic for its stability in organic solvents [38] . As a supporting proof, the weight of the membrane remains stable after being soaked in organic solvents for 24 h ( Supplementary Fig. 5 ). In addition to the thermodynamic stability, yet it is also noticed that ionic bonding is commonly recognized as a dynamic bonding, whereas the rate of bonding exchange is mainly determined by the ionic strength and the state of the material [39] . For example, it has been known that fluid-like polyelectrolyte complexes (for example, complex coacervates, highly swollen gel and so on) undergo appreciable ionic bonding relaxation proportional to the ionic strength. In this study, the membrane actuator is utilized in organic vapours free of additional salts. In this case, the ionic bonding in the membrane is largely alleviated from the relaxation and/or exchanging ( Supplementary Fig. 6 ), which helps maintaining the gradient structures and endurable actuation as will be seen in later sections. Moreover, the as-prepared membranes also feature an interconnected porous architecture (pore size: 200 nm~3 μm) across the membrane ( Fig. 1b–d ). The process of pore formation that we propose ( Supplementary Note 1 ) is related to phase separation of hydrophobic PILTf 2 N in contact with water that creates the pore walls ( Supplementary Fig. 7 ), while the simultaneous electrostatic complexation between PILTf 2 N and C-pillar[5]arene finally builds up the ionic network to stabilise the pore structures ( Supplementary Fig. 8 ) [40] . Superfast actuation of the membrane The PILTf 2 N/C-pillar[5]arene membrane exhibits an unprecedented fast actuation speed in response to acetone stimulus. When placed in acetone vapour (24 kPa, 20 °C), the flat membrane bent quickly into a closed loop in ~0.1 s with the top surface inwards, and further into a multiply wound coil in 0.4 s ( Fig. 2a and Supplementary Movie 1 ). Upon exposure back in air, the membrane recovered its original shape rapidly in ~3 s; this process is reversible and repeatable ( Supplementary Fig. 9 ). The kinetics of the bending and unbending movements is assessed by plotting the curvature of the membrane against time ( Fig. 2b ), resulting in a bending curvature of 1.33 mm −1 in 0.4 s, that is, the 20-mm long membrane actuator bent one complete circle in about every 0.1 s. We compared the actuation speed of the membrane actuator with previously reported polymeric actuators in the literature ( Fig. 2c ). As curvature of bending scales inversely with membrane thickness [41] , we plot ‘curvature × membrane thickness’ versus time, and the lines of constant actuation speed. The fastest actuators are found in the top left of this diagram (red, solid circle). It is seen that our membrane actuator outperforms conventional polymer actuators in terms of the response rate and the amplitude of movement—allowing for the simultaneous combination of ultra-fast actuation and large-scale deformation that existing soft actuators do not exhibit. 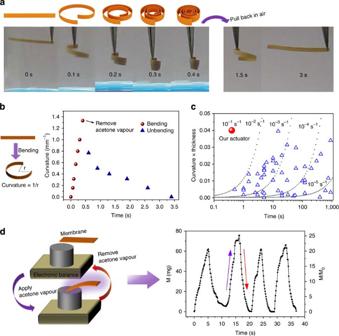Figure 2: Actuation of the membrane actuator. (a) Adaptive movement of a PILTf2N/C-pillar[5]arene membrane (1 mm × 20 mm × 30 μm) placed in acetone vapour (24 kPa, 20 °C, left) and then back in air (right). Note: acetone solvent is stained in blue. (b) Plot of curvature against time for the membrane actuator in (a); on the left: a schematic of how the curvature is calculated. (c) Plot of ‘curvature × thickness’ against time for the membrane actuator in (a) and from literature results (blue triangle) compared with lines of constant actuation speed (Supplementary Fig. 11andSupplementary Table 1). (d) Plot of the force generated by membrane actuator in (a) against time when the membrane was exposed to acetone vapour (24 kPa, 20 °C) and air alternatively;Mis the force that the actuator exerted on the balance;M0is the weight of the actuator membrane. On the left: schematic illustration of the experimental force measurement set-up. Figure 2: Actuation of the membrane actuator. ( a ) Adaptive movement of a PILTf 2 N/C-pillar[5]arene membrane (1 mm × 20 mm × 30 μm) placed in acetone vapour (24 kPa, 20 °C, left) and then back in air (right). Note: acetone solvent is stained in blue. ( b ) Plot of curvature against time for the membrane actuator in ( a ); on the left: a schematic of how the curvature is calculated. ( c ) Plot of ‘curvature × thickness’ against time for the membrane actuator in ( a ) and from literature results (blue triangle) compared with lines of constant actuation speed ( Supplementary Fig. 11 and Supplementary Table 1 ). ( d ) Plot of the force generated by membrane actuator in ( a ) against time when the membrane was exposed to acetone vapour (24 kPa, 20 °C) and air alternatively; M is the force that the actuator exerted on the balance; M 0 is the weight of the actuator membrane. On the left: schematic illustration of the experimental force measurement set-up. Full size image Next, we quantified the mechanical force generated by the membrane bending. As depicted in Fig. 2d , a flat membrane piece was located 2 mm above a cylinder on an electronic balance. When an acetone atmosphere was applied, the membrane bent down towards the cylinder and simultaneously imposed a force on the balance; by cutting off the acetone vapour flow, the original shape was resumed, accompanied by a decrease in the force exerted on the balance. The force was read out directly from the balance in the form of weight (experimental error: 2 mg); it increased and declined rapidly in ~2 and 5 s ( Fig. 2d ), which is coupled to the bending and stretching movements of the membrane actuator towards the on/off state of the acetone vapour. The maximum force detected here (0.75 mN, 75 mg) is already 25 times of the actuator weight (3 mg). In a control experiment without the membrane actuator, only negligible forces can be observed (<1 mg, Supplementary Fig. 10 ). Robustness and multiple responsiveness of the actuator In addition to operation under normal conditions, the actuator survives very harsh treatments. After storage in liquid nitrogen (~−190 °C, 2 h) followed by annealing (150 °C, 24 h) and high-pressure pressing (100 MPa, 24 h), the actuator remained active; it bent into a semicircle in ~0.5 s ( Fig. 3a ), slower than the original form but still significantly faster in comparison with most common polymer actuators ( Fig. 2c ). Morphological examination by scanning electron microscopy (SEM) and porosity analysis by mercury intrusion confirm that partial pore compaction occurs as a result of the high-pressure pressing, which blocks a part of the pore channels ( Supplementary Fig. 12 ) and leads to a slower response rate. Even after a hydrothermal processing (200 °C, 24 h, Supplementary Fig. 13 ), the actuator remained viable ( Fig. 3b ), but the responding rate is 2–3 orders of magnitudes slower possibly due to the enhanced structural relaxation of the ionic bonds and partial degradation. Moreover, the membrane actuator was found to be active in liquid acetone solvent at −50 °C ( Supplementary Fig. 14 ), a temperature well below the glass transition of even most rubbers in which gel-based actuators no longer operate. Aside from this robustness, the smart responsiveness can be rendered to even cylindrical objects by coating the membrane onto them, which is easy to implement owing to the high polarizability and interfacial activity of poly(ionic liquid)s [40] . This possibility is exemplified here by a human hair, which after constructing an asymmetrical coating of the responsive porous membrane onto its surface ‘dances’ in acetone vapour ( Fig. 3c , Supplementary Movie 2 and Supplementary Fig. 15 ). In addition, the membrane actuator also features multi-responsive properties as it readily exhibits hygroscopic actuation. When shaped as a star, the hygroscopic actuator can mimic an ‘artificial flower’ that blossoms and closes in response to humidity changes, indicative of an ability of cooperative actuation to ‘enwrap’ objects ( Fig. 3d ). As such, the actuation spans from the dry state to wet state ( Supplementary Figs 16 and 17 ), which is beneficial because traditional gels usually become inactive when dried. 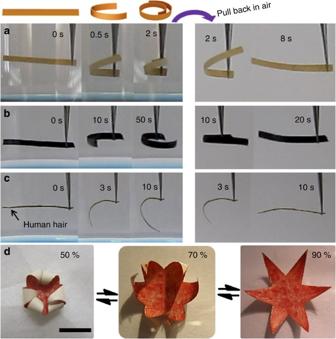Figure 3: Robustness and multiple responsiveness of the actuator. (a) Adaptive movement of a PILTf2N/C-pillar[5]arene membrane (1 mm × 20 mm × 30 μm) placed in acetone vapour (24 kPa, 20 °C, left) and then back in air (right); the membrane was immersed in liquid nitrogen (2 h), followed by annealing (150 °C, 24 h) and high-pressure pressing at 100 MPa for 24 h. (b) The same actuation experiment after hydrothermal processing the membrane in water (200 °C, 24 h). Here the membrane is black owing to its partly carbonaceous nature. (c) Motion of a membrane-coated human hair in acetone vapour and then back in air. (d) The reversible closing and opening of a star-shaped membrane actuator ‘flower’ upon switching the humidity between 50 and 90% at 20 °C; here the top surface of the membrane was stained red while the bottom surface retains the original light yellow colour; inserted number is the relative humidity; scale bar, 1 cm. Figure 3: Robustness and multiple responsiveness of the actuator. ( a ) Adaptive movement of a PILTf 2 N/C-pillar[5]arene membrane (1 mm × 20 mm × 30 μm) placed in acetone vapour (24 kPa, 20 °C, left) and then back in air (right); the membrane was immersed in liquid nitrogen (2 h), followed by annealing (150 °C, 24 h) and high-pressure pressing at 100 MPa for 24 h. ( b ) The same actuation experiment after hydrothermal processing the membrane in water (200 °C, 24 h). Here the membrane is black owing to its partly carbonaceous nature. ( c ) Motion of a membrane-coated human hair in acetone vapour and then back in air. ( d ) The reversible closing and opening of a star-shaped membrane actuator ‘flower’ upon switching the humidity between 50 and 90% at 20 °C; here the top surface of the membrane was stained red while the bottom surface retains the original light yellow colour; inserted number is the relative humidity; scale bar, 1 cm. Full size image Actuation mechanism The mechanism for this unique actuation is addressed at two levels: why the membrane could bend in response to acetone vapour, and what is the key structure responsible for the superfast bending kinetics ( Fig. 4 ). 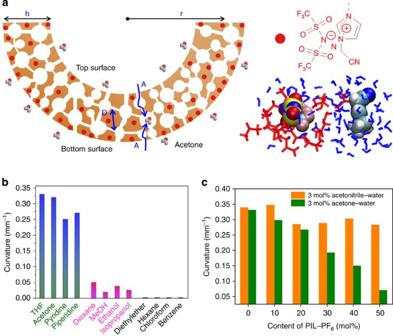Figure 4: Actuation mechanism via solvent molecule sorption. (a) A scheme of the porous membrane actuator (left, not to scale), definition of variables:h, thickness of the membrane;r, radius of the bended membrane arch;D, thickness of the pore wall;A, the diffusion track of acetone molecules from outside to the surface of pore walls inside the membrane; (top right) chemical structure of the ‘imidazolium~Tf2N’ pair; (lower right) the representative snapshot of solvent redistribution around the ‘imidazolium ~ Tf2N’ ion pair: water molecules (blue) are partially displaced by acetone molecules (red), which adsorb more to the Tf2N anion on the left of the snapshot. (b) Curvatures of PILTf2N/C-pillar[5]arene membrane actuator in vapour of different solvents (2 kPa, 20 °C). (c) Effect of PF6anion content on curvature of PIL(Tf2N+PF6)/C-pillar[5]arene membrane actuator in 3 mol% acetonitrile–water and 3 mol% acetone–water mixture, respectively. First, from a purely geometric perspective the curvature C =1/ r scales as Figure 4: Actuation mechanism via solvent molecule sorption. ( a ) A scheme of the porous membrane actuator (left, not to scale), definition of variables: h , thickness of the membrane; r , radius of the bended membrane arch; D , thickness of the pore wall; A , the diffusion track of acetone molecules from outside to the surface of pore walls inside the membrane; (top right) chemical structure of the ‘imidazolium~Tf 2 N’ pair; (lower right) the representative snapshot of solvent redistribution around the ‘imidazolium ~ Tf 2 N’ ion pair: water molecules (blue) are partially displaced by acetone molecules (red), which adsorb more to the Tf 2 N anion on the left of the snapshot. ( b ) Curvatures of PILTf 2 N/C-pillar[5]arene membrane actuator in vapour of different solvents (2 kPa, 20 °C). ( c ) Effect of PF 6 anion content on curvature of PIL(Tf 2 N+PF 6 )/C-pillar[5]arene membrane actuator in 3 mol% acetonitrile–water and 3 mol% acetone–water mixture, respectively. Full size image where ε b and ε t are the swelling strains due to ‘solvent~membrane’ interactions in the bottom and top regions, respectively, and h is the membrane thickness [41] . Any stimulus that can drive the actuator must be able to impact ε b and ε t unequally. In line with the definition of DEC ( Fig. 1c and Supplementary Fig. 4 ), a part of imidazolium units from PILTf 2 N undergoes complexation with C-pillar[5]arene and provides a stable network because C-pillar[5]arene is insoluble in acetone and the electrostatic complexation bonding features high stability in organic solvent ( Supplementary Figs 5 and 6 ) [38] . Meanwhile, the rest of PILTf 2 N is not involved in complexation and exists as ‘imidazolium~Tf 2 N’ ion pairs, shown by the chemical structures in Fig. 4a . The existence and density of the ‘imidazolium~Tf 2 N’ ion pairs are confirmed by monitoring the sulphur content along the cross-section. In this context it is important to note that strong interactions exist between acetone solvent molecules and the ‘imidazolium~Tf 2 N’ ion pair, because the acetone solvent can easily dissolve PILTf 2 N. We conducted atomistically resolved molecular dynamics computer simulations of the ‘imidazolium~Tf 2 N’ pair in water–acetone mixtures to probe the interaction between acetone solvent and ‘imidazolium~Tf 2 N’ ion pair ( Supplementary Note 2 ). Indeed, the simulation reveals that the acetone adsorbs stronger to the ion pair than water ( Supplementary Figs 18–20 ). In particular, a large number of water molecules are preferentially replaced by acetone molecules around the rather hydrophobic fluorine groups of the Tf 2 N anion ( Supplementary Table 2 ), see the molecular dynamics snapshot on the right hand side of Fig. 4a and the analysis ( Supplementary Fig. 20 ). When the membrane is placed in acetone vapour, the solvent molecules diffuse rather rapidly into the porous membrane from both the top and bottom surfaces, as indicated by the blue track ‘A’ schemed in Fig. 4a . The acetone molecules will adsorb to the ‘imidazolium~Tf 2 N’ ion pair (red dots, Fig. 4a ) owing to their preferential interaction with the anion. Given the gradient of DEC along the cross-section (that is, the bottom surface region has more ‘imidazolium~Tf 2 N’ ion pairs owing to the smaller DEC, Fig. 1c ), understandably the bottom surface region is more solvated by acetone compared with the top. As such, the local solvent osmotic pressure increase leads to more swelling [42] of the bottom part, such that ε b >ε t and the membrane bends with the top surface inwards according to equation (1). Of course a complexation gradient will also give rise to a gradient in modulus, which will in turn change the amount of curvature on swelling; this, however, is a second-order effect in comparison to the gradient in swellability [41] . Moreover, equation (1) suggests that, if the mechanical properties are uniform through the thickness, only small swelling strain differences of around 4% would account for the maximum curvature reached of C =1.34 mm −1 . This is in good agreement with the observation that at the maximum bending, the porous morphology of the membrane actuator shows little-to-no detectable change when the experimental error is considered ( Supplementary Fig. 21 ). As another support to this mechanism, it is found that the amplitude of actuation in general is specific and proportional to the ‘solvent~PILTf 2 N’ interaction, if various solvents are compared. For example, the solvents (acetone, THF, piperidine and pyridine, Supplementary Table 3 ) that can dissolve PILTf 2 N polymer, that is, strong ‘solvent~PILTf 2 N’ interactions trigger the strongest actuation ( Fig. 4b ); solvents (dioxane, methanol, ethanol and isopropanol) that cannot dissolve but can swell the PILTf 2 N polymer only drive the actuator with slower kinetics and weaker bending ( Fig. 4b ). On the contrary, solvents that can neither dissolve nor swell the PILTf 2 N polymer (diethyl ether, benzene, cyclohexane and chloroform) fail to drive the actuator, that is, the polymer membrane does not bend at all in the vapour of these solvents. Further evidence is given by the anion effect ( Fig. 4c ): we exchanged the Tf 2 N anion with PF 6 , which has a weak interaction with acetone but strong interaction with acetonitrile (PILPF 6 is insoluble in acetone but soluble in acetonitrile). By exchanging Tf 2 N stepwise with PF 6 anions, the actuation curvature of PIL(Tf 2 N+PF 6 )/C-pillar[5]arene membrane in aqueous acetone solution gradually decreases while that in aqueous acetonitrile basically remains the same. As such, both Fig. 4b and Fig. 4c clearly confirm that the stronger ‘solvent~PILTf 2 N’ interaction on a molecular level produces stronger actuation, which agrees well with the solvent sorption mechanism. Regarding the gradient structures, we prepared a control membrane that has a similar porous morphology but a symmetrical DEC distribution across the membrane ( Supplementary Fig. 22 ). Now, the membrane only slightly bends when placed in acetone vapour, because the actuation stress now on both surfaces largely offsets each other ( Supplementary Note 3 ). With respect to the fast bending kinetics, swelling is a diffusion-determined process in which the rate-determining step is that the solvent molecules have to diffuse through the dense polymer network to reach their final absorption sites. The standard diffusion law is expressed in equation where is the mean squared distance travelled in a time t and γ is the diffusion constant. For a nonporous material, the solvent has to travel a mean distance on the order of the membrane thickness, , to solvate the whole membrane. For our porous membrane with submicron scale interconnected pore channels, the solvent vapour molecules can almost instantaneously travel to the pore surfaces via the unhindered (percolating) micron-sized pore channel access (blue track ‘A’ schemed in Fig. 4a ). Then, the acetone molecules only have to diffuse through a distance of roughly , which is the average thickness of the pore wall, to solvate the whole polymer matrix. From the cross-sectional SEM image in Fig. 1b , the average D is estimated to be <1 μm, which is much smaller than the overall membrane thickness, h =30 μm. Using the diffusion law in equation (2), the diffusion time ratio for porous materials ( t p ) and nonporous materials ( t np ) can be expressed by which indicates that the diffusion rate in the porous membrane is improved by almost three orders of magnitude ( D ~1 μm compared with h ~30 μm, thus ( D/h ) 2 ~1/900). Thus, the porous architecture accelerates the actuation speed by providing an instant access to the pore walls throughout the membrane, and reducing the rate-determining diffusion distance. As a comparison, we prepared another nonporous control membrane that retains the linear gradient ( Supplementary Fig. 23 ); understandably the membrane shows slower responsiveness and smaller bending towards acetone stimulus. Furthermore, we found that the partial pore compaction resulting from the high-pressure pressing (100 MPa) also reduced the actuation kinetics ( Fig. 3a and Supplementary Fig. 12 ), since normally the denser the porous structure is, the slower the diffusion is. Traditionally, the swelling of the polymer networks is the dominant mechanism to modulate hydrogel and ion gel actuators, but it is a relatively slow process limited by the retarded diffusion in the wet state. In our actuator design, a gradient structure was introduced into an electrostatically cross-linked porous membrane, whereas the sorption of the solvent vapour molecules at the pore surface results in a local volume change giving rise to actuation movements. Importantly, due to the pore-accelerated mass transport, the surface sorption can take place instantaneously in contact with solvent vapour molecules, at a speed of three orders of magnitude faster than bulk swelling. As such, the PILTf 2 N/C-pillar[5]arene actuator features an instant, robust and multiple responsiveness spanning both the wet and dry modes. Not only the actuator gives a record actuation speed among all synthetic polymer actuators so far, the combination of multiple advantages in one single actuator sets it apart from previous soft actuators. For example, the membrane appeared responsive even towards vapours from perfume or tea tree oil (both contain a considerable amount of ethanol, Supplementary Movie 3 ), verifying its actuation ability to bio-benign stimuli. More significantly, in line with the actuation mechanism and owing to the actuator’s versatile responsiveness to a variety of organic solvents, the membrane actuator can distinguish 13 types of aqueous miscible solvents through two simple sets of actuation experiments ( Supplementary Fig. 24 ). We regard this implication as substantial because it renders the actuation available for facile and quantitative analysis of solvent quality without the need of sophisticated or expensive instruments ( Supplementary Note 4 ). By further modulating the ‘PIL~solvent’ interactions and the porous morphologies, exciting opportunities may arise as it can foster high throughput analysis with improved resolution and capacity, which is now ongoing in our lab. This conceptual methodology is virtually applicable to a wide range of polymers and small molecules with complementary interactions, opening new avenues for adaptive soft matters with fast response rate and complex movements. In addition, given the ionic nature of the constituent polymers and solution-based processing, the underlying principles seamlessly interface with more fabrication technologies, such as spinning and patterning, holding great promise for micro-actuation devices of high complexity and smart ionics spanning multiple length scales. Materials Lithium bis(trifluoromethanesulfonyl)imide (LiTf 2 N, 99.95%) and concentrated aqueous ammonia (28 wt%) were purchased from Sigma-Aldrich and used without further purification. All organic solvents were of analytic grade. The PILTf 2 N was synthesized according to our previous study [43] . The C-pillar[5]arene was synthesized according to a literature method [44] . Both the PILTf 2 N and C-pillar[5]arene were characterized by 1 H nuclear magnetic resonance measurements (Bruker DPX-400 spectrometer), which were carried out at room temperature using DMSO-d 6 and D 2 O as solvents ( Supplementary Fig. 1 ). The apparent molecular weight and polydispersity index of PCMVImTf 2 N polymer was 1.15 × 10 5 g mol −1 and 2.95, respectively. All the solvents used in this study were of analytic grades. Preparation and characterization of membrane actuators Typically, 1.0 g of PILTf 2 N polymer and 0.27 g of C-pillar[5]arene were dissolved in 10 ml of DMSO solvent to form a homogeneous solution. Then the solution was cast onto a clean glass plate, dried at 80 °C for 1 h and soaked in 0.2 wt% aqueous ammonia (2 h, 20 °C), giving rising to free-standing membranes with thickness ~30 μm. Note that membrane actuators can be modulated by tailoring the concentration of ammonia (0.02~0.2 wt%) and the soaking time (2~48 h). Morphologies of the membranes were examined by SEM performed on a GEMINI LEO 1550 microscope at 3 kV; samples were coated with a thin layer of gold before examination. The porosity of the membrane was measured by mercury intrusion porosimeter for meso- and macropore analysis (Autopore III, Micromeritics USA, DIN 66133) at BAM Federal Institute for Materials Research and Testing, Berlin. To measure the sulphur content along the membrane cross-section, a porous membrane (thickness ~100 μm) was prepared and the elemental composition at different positions along the membrane cross-section was analysed by means of energy dispersive X-ray (EDX, Oxford instruments) via SEM ( Supplementary Fig. 4 ). Solvent vapour stimulus actuation Organic solvents were put in a glass beaker at 20 °C. Then a piece of membrane strip (20 mm × 1 mm × 30 μm) was placed ~5 mm above the liquid phase of the solvent; the solvent vapour will trigger the fast bending movement. Afterwards, the membrane was pulled back into air to accomplish the shape recovery. This process was repeated for 50 times to confirm the good durability of the actuation function. For the perfume-triggered actuation, perfume (Coco Mademoiselle, Chanel) was used instead of organic solvents. Please note: in all cases, the membrane actuator was NOT in contact with the liquid body of both the solvents and perfume. All the actuation movements were recorded by a digital camera (Canon IXUS130, frames per second: 30). For hygroscopic actuation ( Fig. 3d ), the star-shaped membrane (30 μm thick) was placed in a test chamber (model WKL 34, Weiss Technik), whereby the temperature was kept 20 °C and the relative humidity was modulated from 50% to 90%, during which the membrane flow open and closed reversibly. How to cite this article: Zhao, Q. et al. An instant multi-responsive porous polymer actuator driven by solvent molecule sorption. Nat. Commun. 5:4293 doi: 10.1038/ncomms5293 (2014).